Conflict acts as an implicit cost in reinforcement learning Conflict has been proposed to act as a cost in action selection, implying a general function of medio–frontal cortex in the adaptation to aversive events. Here we investigate if response conflict acts as a cost during reinforcement learning by modulating experienced reward values in cortical and striatal systems. Electroencephalography recordings show that conflict diminishes the relationship between reward-related frontal theta power and cue preference yet it enhances the relationship between punishment and cue avoidance. Individual differences in the cost of conflict on reward versus punishment sensitivity are also related to a genetic polymorphism associated with striatal D1 versus D2 pathway balance (DARPP-32). We manipulate these patterns with the D2 agent cabergoline, which induces a strong bias to amplify the aversive value of punishment outcomes following conflict. Collectively, these findings demonstrate that interactive cortico–striatal systems implicitly modulate experienced reward and punishment values as a function of conflict. Motivated action selection is effortful, and often occurs during difficult or challenging circumstances. These coincident descriptors all share a common theme of being energetically expensive, and thus they are all likely to be avoided. Increasing evidence suggests that effortful control of this sort diminishes the value of state-action selection by adding expense to a cost/benefit computation in cortico–striatal circuits. Similar to effort, conflict monitoring has recently been proposed to register as a cost [1] , particularly mediated by midcingulate cortex (MCC). Yet, existing empirical support for MCC involvement in conflict costs have largely relied upon explicit manipulations of cognitive effort, and not conflict per se [2] , [3] , [4] , [5] . While some studies have demonstrated aversion-inducing effects of response conflict, these studies did not examine the neural mechanisms by which this effect is instantiated [2] , [6] , [7] . Here we demonstrate that response conflict acts as a cost during reinforcement learning by both diminishing reward value and boosting punishment aversion. Moreover, we provide evidence that the extent to which conflict modulates reinforcement value relates to MCC responses to conflict as well as downstream striatal dopaminergic valuation. While MCC registers effort costs, a cost/benefit computation appears to be reflected by a diminishment of positive prediction error signalling in ventral striatum [3] , [8] , [9] , [10] . In fact, striatal dopamine has been particularly implicated in the cost of effort. A greater willingness to expend effort is related to increased striatal dopaminergic tone [11] , [12] and can be induced with dopamine agonism [13] , [14] . Conversely, dopamine depletion or antagonism diminishes the willingness to trade effort for reward [14] , [15] , [16] . Structurally, D2 receptor overexpression shifts the cost/benefit calculation towards greater cost [17] , [18] . Collectively, these findings suggest distinct roles of MCC, striatal dopaminergic receptors and striatal dopaminergic tone in determining the cost of effort. These findings provide a methodological scaffolding to examine if response conflict affects these systems in a manner similar to effort. Here we aimed to assess and manipulate the functioning of these distributed systems in humans during a learning task with separate conditions associated with varying degrees of response conflict. To quantify MCC activities, we monitored the electroencephalography (EEG) feature of frontal midline theta (FMθ). FMθ has been suggested to operate as a common mechanism for MCC operations to events, indicating a need for control (for example, effort, conflict, punishment and error; refs 19 , 20 ). These types of aversive events contribute to avoidance and behavioural inhibition, which can reliably be predicted by FMθ amplitude [21] . Individual differences in striatal dopamine related to reinforcement learning were assessed by genotyping a genetic polymorphism affecting the relative influence of competing action selection pathways (D1 versus D2). Dopamine bursts in the cortico–striatal D1 direct pathway underlies ability to learn from and seek reward, whereas dopamine dips in the D2-mediated indirect pathway underlies the ability to learn from and avoid punishment [22] , [23] , [24] , [25] . Computational models show how the striatal D1 and D2 pathways come to represent values and costs in such tasks, and that choices in reward-based tasks are best described by an opponent process whereby each choice option has a corresponding positive (D1) and negative (D2) action value [26] . The dopamine- and cyclic AMP-regulated phosphoprotein (DARPP-32) has been used as a marker for cortico–striatal plasticity, where an increasing number of T alleles predict an imbalance in learning favouring D1 relative to D2 pathways. DARPP-32 levels in rat NAcc predicts a shift towards greater willingness to exert effort for reward [15] and individual differences in human DARPP-32 T alleles predict the ability to learn from reward [27] , [28] , [29] . Finally, we assessed the potential causal role for dopaminergic function in conflict-related learning biases by administering low dose of cabergoline in a double blind pharmacological challenge. Low doses of cabergoline tend to preferentially stimulate pre-synaptic D2 autoreceptors, which specifically inhibit phasic dopamine bursts in the striatum. Previous studies have shown that low doses of D1 agonists decrease reward learning and consequently increase relative learning from punishment, whereas low doses of D2 antagonists have the opposite effect [30] , [31] , [32] , [33] . To track individual differences in the outcome of this pharmacological manipulation, we measured spontaneous eye blink rate, thought to be a correlate of striatal dopaminergic tone [34] , [35] , [36] , [37] . In this series of experiments, we aimed to test the theoretically motivated hypothesis that conflict acts as a cost during reinforcement learning and action selection [1] . Using a tightly controlled novel task, Study I capitalized on previously validated measures of cortical (FMθ) and striatal (DARPP-32) systems that contribute to individual differences in reinforcement learning, whereas Study II directly manipulated dopamine activity (cabergoline challenge) and monitored individual differences in this response via dopaminergic correlates (eye blinks). Collectively, these findings provide multiple independent lines of evidence to suggest that response conflict acts as a cost to diminish reward value and enhance punishment aversion within an integrated cortico–striatal circuit. Study I participants and task A total of 83 adults were recruited from the Brown University undergraduate subject pool and Providence community to complete the experiment (mean age=20 years, range=18–30 years, 52 female). Samples of saliva (~4 cc) were obtained from each subject using the Oragene system (DNA Genotek). A novel task was created to elicit response conflict during a reinforcement learning task (training phase) and subsequently assess the influence of conflict on learning (testing phase). After a brief practice period, participants each performed six training–testing blocks. Data were averaged together across all blocks for analysis. In each training phase, a modified Simon [38] task was utilized to elicit response conflict during the presentation of four unique stimuli ( Fig. 1a,b ). Each stimulus was presented to the left or right side of the screen. Participants were instructed to press the left game pad button when the stimulus was yellow and the right button when it was blue. These presentations were thus either spatially congruent (screen side=response hand) or incongruent (screen side≠response hand) as in a standard Simon task. Stimuli consisted of four randomly assigned unique shapes (termed ‘A’, ‘B’, ‘C’ and ‘D’). Following an accurate response, participants experienced a constant 170 ms delay followed by the presentation of reinforcement feedback (1,000 ms duration) where they could gain points (rewarded trial; +1) or not (punishing trial; 0) according to a probabilistic schedule described below. Although these points were not relevant for learning the Simon rule contingencies (which again were instructed), participants were informed that some stimuli would be more often rewarding than others and that they should learn which ones were better so they could identify them after the training block. 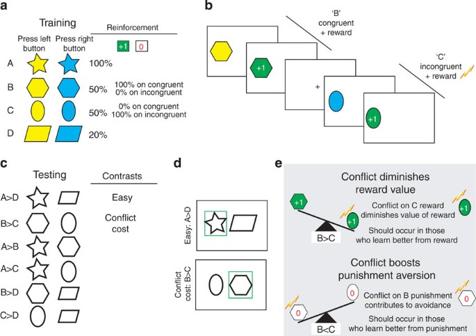Figure 1: Task dynamics and hypothesized effects of the cost of conflict. (a,b) In the training phase, four different stimuli were associated with different reinforcement probabilities. The manipulation of the cost of conflict utilized preferential reinforcement for the B and C stimuli, where B was only rewarded following congruent Simon presentations (for example, yellow on left) and C was only rewarded following incongruent Simon presentations that induce response conflict (for example, blue on left), indicated here by the lightning bolt. (c,d) In a subsequent testing phase, participants had to choose the ‘most rewarding’ stimulus in a two alternative forced-choice scenarios. Separate contrasts were used to aggregate test phase selections. The easy condition assessed basic performance: the ability to select the best option over the worst option (A>D). The influence of congruency-reinforcement pairings assessed the conflict cost contrast (B>C). (e) Hypothesized effects of the cost of conflict during training on action selection during the testing phase. Rewards followed conflict in the C condition, which was hypothesized to diminish the relative value of reward for C versus B, leading to greater selection of B in the test phase. Punishments followed conflict in the B condition, which was hypothesized to increase the effect of punishment for B versus C, learning to greater avoidance of B in the test phase. Thus, any aggregate bias for B>C or C>B should be contingent on individual differences in learning from reward or avoiding punishment, which have previously been characterized using EEG, genetics and dopamine pharmacology. Figure 1: Task dynamics and hypothesized effects of the cost of conflict. ( a , b ) In the training phase, four different stimuli were associated with different reinforcement probabilities. The manipulation of the cost of conflict utilized preferential reinforcement for the B and C stimuli, where B was only rewarded following congruent Simon presentations (for example, yellow on left) and C was only rewarded following incongruent Simon presentations that induce response conflict (for example, blue on left), indicated here by the lightning bolt. ( c , d ) In a subsequent testing phase, participants had to choose the ‘most rewarding’ stimulus in a two alternative forced-choice scenarios. Separate contrasts were used to aggregate test phase selections. The easy condition assessed basic performance: the ability to select the best option over the worst option (A>D). The influence of congruency-reinforcement pairings assessed the conflict cost contrast (B>C). ( e ) Hypothesized effects of the cost of conflict during training on action selection during the testing phase. Rewards followed conflict in the C condition, which was hypothesized to diminish the relative value of reward for C versus B, leading to greater selection of B in the test phase. Punishments followed conflict in the B condition, which was hypothesized to increase the effect of punishment for B versus C, learning to greater avoidance of B in the test phase. Thus, any aggregate bias for B>C or C>B should be contingent on individual differences in learning from reward or avoiding punishment, which have previously been characterized using EEG, genetics and dopamine pharmacology. Full size image The four stimuli had different reinforcement rates: the ‘A’ stimulus was 100% rewarding and the ‘D’ stimulus was 20% rewarding, each consisting of an equal number of rewards on congruent versus incongruent trials (and also on yellow versus blue colours and left versus right sides). In contrast, while stimuli B and C were equivalently reinforced at 50% rates each, the ‘B’ stimulus was reinforced on 100% of congruent trials and 0% of incongruent trials, whereas the ‘C’ stimulus was reinforced on 0% of the congruent trials and 100% of the incongruent trials. Thus if conflict reduces the value of rewards, it should reduce the learned positive value of C relative to B; conversely, if it amplifies the aversive value of negative outcomes it should cause B to have a more negative value than C. Note that B and C stimuli were also equally reinforced for each yellow and blue occurrence and in left and right locations; the sole difference between them was in the consistent experience of conflict prior to reward (‘C’) or punishment (‘B’). If participants did not respond by the response time (RT) deadline (1,000 ms) or if they made an error, they received informative feedback (‘No Response’ or ‘ERROR!’) and the same trial was immediately repeated. This yielded a deterministic reinforcement schedule for each stimulus within each block: participants always experienced the exact reinforcement schedule regardless of errors or delays. There were 20 occurrences of each stimulus per training block. The inter-trial interval consisted of a fixation cross for 1,000 ms. Following each training phase, participants entered a forced-choice testing phase where they were instructed to select ‘the most rewarding’ stimulus from each unique pair of stimuli (each pair occurred four times=48 trials total, 3,000 ms response deadline, Fig. 1c,d ). This testing phase provided the critical assessment of biased reinforcement learning. First, it was expected that participants should be able to reliably select A>D, this was termed the ‘Easy’ contrast. In contrast, the B versus C choice was denoted the ‘conflict cost’ contrast. As noted above stimuli B and C were equally reinforced at 50% rates, but the degree to which participants reliably selected B>C is a measure of the extent to which conflict acted to diminish the reward value of C, and hence subjects making choices primarily based on reward should prefer B to C. Conversely, the degree to which they select C>B is indicative of conflict acting to enhance the aversive value of B. Individuals with aggregate conflict cost contrast values higher than chance (0.5) showed a bias to favour B>C and vice versa for values lower than chance. Figure 1e explicitly details the two ways that conflict could influence such reinforcement biases: conflict could diminish the value of reward (on ‘C’ specifically, leading to a B>C bias) or boost the impact of punishment (on ‘B’ specifically, leading to a C>B bias). Thus the perfectly crossed design eliminates any chance of performance bias due to task demands unrelated to conflict, but it also obviates an assessment of an aggregate conflict effect on choice preferences. Study I tested the hypothesis that the bias to choose B over C or vice versa would depend on individual differences in two moderators previously shown to predict reward versus punishment learning: (1) electrophysiological markers of the salience of positive and negative outcomes in MCC [39] , [40] and (2) striatal dopaminergic function in D1 versus D2 systems [27] , [28] . Study I performance During training, participants had an average error rate of 5% (s.d.=3%), with an average congruent RT of 574 ms and a small but significant 12 ms delay due to conflict (incongruent >congruent t 82 =4.04, P =1.2 e−4 , Fig. 2a , Supplementary Fig. 1 ). During testing, participants were nearly perfect when selecting A>D in the easy contrast (95% accuracy), and had no main effect of a conflict cost bias in accuracy due to conflict ( t -test against chance <1, Fig. 2b ). However this absence of population effect does not imply a null effect of the task manipulation; box plots reveal a considerable range of scores across individuals. It was specifically hypothesized that this inter-individual variance would be accounted for by the tendency for participants to associate conflict to reward or to punishment based on predictable individual differences as described above. 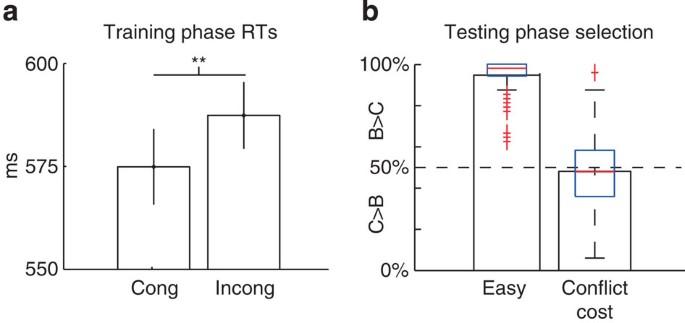Figure 2: Study I performance. (a) training phase RT: at-test (N=83) revealed a significant conflict effect in RT during Simon task performance. (b) testing phase accuracies: while participants were nearly perfect in selecting A>D in the easy condition, there was no evidence for a global effect of a conflict cost bias. However, box plots demonstrate considerable inter-individual differences in these measures of bias. Error bars are mean ±s.e.m. **P<0.01. Figure 2: Study I performance. ( a ) training phase RT: a t -test ( N =83) revealed a significant conflict effect in RT during Simon task performance. ( b ) testing phase accuracies: while participants were nearly perfect in selecting A>D in the easy condition, there was no evidence for a global effect of a conflict cost bias. However, box plots demonstrate considerable inter-individual differences in these measures of bias. Error bars are mean ±s.e.m. ** P <0.01. Full size image Study I EEG EEG data from the training phase was investigated to determine if the common FMθ feature of conflict and punishment was related to biased action selection in the testing phase. EEG was recorded on a 64-channel Brain Vision system, then subsequently pre-processed (See Online Methods) and converted to current source density [41] . Time–frequency calculations were computed using custom-written Matlab routines (see Methods). 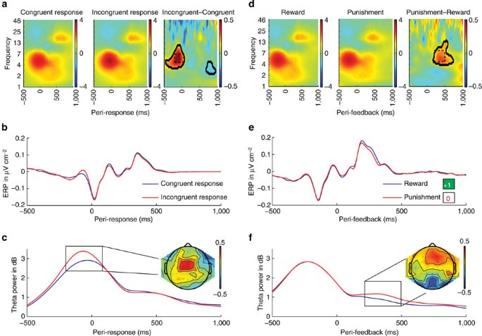Figure 3: Training phase EEG (FCz electrode) to conflict and feedback, demonstrating a common theta band burst to conflict and punishment. (a) Time-frequency plots of responses highlight a significant effect of pre-response theta power to conflict (t-tests,N=83), indicated by black contours in the difference plot. A Region-of-Interest (ROI) was identified from −200 to 50 ms peri-response in the 4–8 Hz range (dotted box). (b) ERPs showed a larger pre-response modulation due to conflict. (c) The time course of theta power within the ROI shows that conflict-related effects were maximal over mid-frontal regions. (d) Time–frequency plots of feedbacks highlight a significant effect of post-feedback theta power to punishment. An ROI was identified from 200–500 ms post-feedback in the 4–8 Hz range. (e) ERPs show a feature of a reward-related slow positivity, which obscures many of the theta band dynamics revealed by spectral analyses. (f) The time course of theta band power within the ROI shows that punishment-related theta band enhancement was maximal over anterior mid-frontal regions. Figure 3 shows the expected theta band enhancements to conflict and feedback at the FCz (mid-frontal) electrode. Conflict was associated with significantly enhanced pre-response theta power ( Fig. 3a ) and event-related potential (ERP) amplitude ( t 82 =4.40, P =3.3 e−5 , Fig. 3b ). The topographical distribution of this conflict-related theta power differential was maximal over mid-frontal electrodes ( Fig. 3c ). Reward and punishment were associated with relatively small modulations in overall spectral power compared with the response-related activities, yet there was an expected significant difference with punishment conditions causing relatively greater theta power than reward ( Fig. 3d ). The ERP following feedback mainly consisted of a slowly decaying slope, with reward having higher amplitude than punishment ( t 82 =6.74, P =2 e−9 , Fig. 3e ). This effect was due to greater delta band phase consistency for reward, consistent with ideas of a reward-related posterior positivity in the delta band [19] , [42] ( Supplementary Fig. 2 ). The non-phase locked theta band power difference was largest in anterior midline sites ( Fig. 4f ). Collectively, these findings demonstrate expected frontal theta band power enhancements to conflict and punishment, in line with the suggestion that FMθ reflects a common MCC mechanism for adaptation to salient and aversive events [19] , [20] . Figure 3: Training phase EEG (FCz electrode) to conflict and feedback, demonstrating a common theta band burst to conflict and punishment. ( a ) Time-frequency plots of responses highlight a significant effect of pre-response theta power to conflict ( t -tests, N =83), indicated by black contours in the difference plot. A Region-of-Interest (ROI) was identified from −200 to 50 ms peri-response in the 4–8 Hz range (dotted box). ( b ) ERPs showed a larger pre-response modulation due to conflict. ( c ) The time course of theta power within the ROI shows that conflict-related effects were maximal over mid-frontal regions. ( d ) Time–frequency plots of feedbacks highlight a significant effect of post-feedback theta power to punishment. An ROI was identified from 200–500 ms post-feedback in the 4–8 Hz range. ( e ) ERPs show a feature of a reward-related slow positivity, which obscures many of the theta band dynamics revealed by spectral analyses. ( f ) The time course of theta band power within the ROI shows that punishment-related theta band enhancement was maximal over anterior mid-frontal regions. 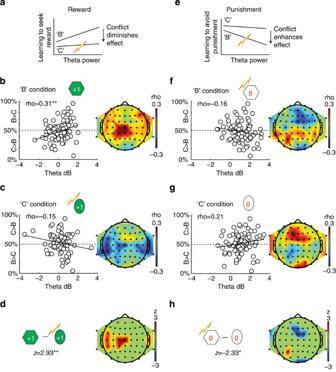Figure 4: EEG reveals evidence for cortical systems (FMθ) affected by the cost of conflict during both diminished reward value and enhanced punishment aversion. The topography of correlation coefficients (FMθ and choice bias) is shown for each empirical contrast, as well as a scatterplot from the identified electrode on each topomap. (a) In the case of rewarding feedback, conflict was hypothesized to diminish the relationship between salience of reward and future action selection. (b) Individuals with greater reward-related theta on the B condition had a stronger bias to seek B>C. (c) Individuals with greater reward-related theta on the C condition (following conflict) had no relationship between feedback-related activities and action selection. (d) The difference between reward-related correlation coefficients was significant in mid-frontal areas, demonstrating how the conflict diminished the relationship between reward-related cortical signals and action valuation. (e) In the case of punishing feedback, conflict was hypothesized to enhance the relationship between salience of losses and future action avoidance. (f) Individuals with greater punishment-related theta on the B condition (following conflict) had a non-significant bias to avoid B (C>B bias). (g) Individuals with greater punishment-related theta on the C condition had an inverse, non-significant relationship between punishment-related activities and action avoidance. (h) The difference between punishment-related correlation coefficients was significant in anterior mid-frontal areas, demonstrating that conflict boosted the relationship between punishment-related cortical signals and action avoidance. Correlations were Spearman’s rho tests (N=83),zindicates rho-to-z-test of differences between coefficients. *P<0.05; **P<0.01. Full size image Figure 4: EEG reveals evidence for cortical systems (FMθ) affected by the cost of conflict during both diminished reward value and enhanced punishment aversion. The topography of correlation coefficients (FMθ and choice bias) is shown for each empirical contrast, as well as a scatterplot from the identified electrode on each topomap. ( a ) In the case of rewarding feedback, conflict was hypothesized to diminish the relationship between salience of reward and future action selection. ( b ) Individuals with greater reward-related theta on the B condition had a stronger bias to seek B>C. ( c ) Individuals with greater reward-related theta on the C condition (following conflict) had no relationship between feedback-related activities and action selection. ( d ) The difference between reward-related correlation coefficients was significant in mid-frontal areas, demonstrating how the conflict diminished the relationship between reward-related cortical signals and action valuation. ( e ) In the case of punishing feedback, conflict was hypothesized to enhance the relationship between salience of losses and future action avoidance. ( f ) Individuals with greater punishment-related theta on the B condition (following conflict) had a non-significant bias to avoid B (C>B bias). ( g ) Individuals with greater punishment-related theta on the C condition had an inverse, non-significant relationship between punishment-related activities and action avoidance. ( h ) The difference between punishment-related correlation coefficients was significant in anterior mid-frontal areas, demonstrating that conflict boosted the relationship between punishment-related cortical signals and action avoidance. Correlations were Spearman’s rho tests ( N =83), z indicates rho-to- z -test of differences between coefficients. * P <0.05; ** P <0.01. Full size image Study I feedback theta predicts action selection biases We hypothesized that the degree to which conflict modulated reward- and punishment-related theta activity during training would relate to choice preferences at test. Figure 4 shows the inter-individual correlations between training phase stimulus-specific feedback-locked theta power and test phase preferences. Relative reductions in reward-related theta power to C (characterized by conflict) compared with B were suggested to predict an increased preference for B over C ( Fig. 4a ). This hypothesis was supported by significant differences in the coefficients linking cortical midline theta to choice preferences during rewards following the B versus C conditions, as revealed by a rho-to- z test ( Fig. 4d : z 82 =2.93, P =3 e−3 ). This was further substantiated by a simple effect whereby greater theta following rewards in the B condition was related to greater preferences for B over C (rho 81 =0.31, P =5 e−3 ), whereas this relationship was absent in the C condition that was characterized by reward-related conflict (rho 81 =−0.15, P =0.19), see Fig. 4b–c . Conversely, we hypothesized that conflict should enhance the relationship between punishment-locked theta power in training and stimulus avoidance at test ( Fig. 4e ). Indeed, theta power during punishments following B versus C was differentially predictive of subsequent B versus C test choices ( Fig. 4h : z 82 =−2.33, P =0.02), with opposite numerical trends in each condition (B: rho 81 =−0.16, P =0.15; C: rho 81 =0.21, P =0.06; Fig. 4f,g ). To clarify and extend these findings, we also looked at posterior delta band activities after feedback, which have been suggested to specifically relate to rewards [42] , unlike feedback-locked FMθ which primarily reflects feedback salience and not valence per se [43] , [44] . Supplementary Figure 3 demonstrates a similar pattern of correlations to Fig. 4a–d but in posterior delta during reward (with no effects for punishment). In sum, the degree to which conflict reduced reward-related theta/delta activity of C compared with B was related to preferences for B, and the degree to which conflict enhanced punishment-related theta activity of B compared with C was related to avoidance of B. These findings suggest that conflict acted to both diminish reward value and to boost punishment avoidance within cortical systems associated with interpreting the salience of feedback. 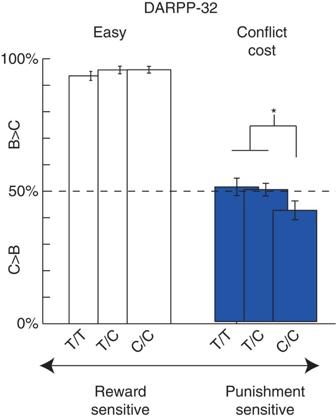Figure 5: A genetic polymorphism in dopamine receptors predicted individual differences in the cost of conflict on reward versus punishment. The presence of a DARPP-32 C allele was associated with an increased C>B bias in the conflict cost contrast (t-test,N=83), bolstering the hypothesis that conflict diminished reward value (on the C stimulus) more in individuals biased to learn from reward and boosted punishment aversion (on the B stimulus) more in those biased to learn from punishment. Error bars are mean±s.e.m. *P=0.05. Study I genetics Figure 5 shows the effects of individual differences in the genetic polymorphism for DARPP-32, which primarily affects striatal dopaminergic functioning associated with D1 and D2 pathways related to learning from positive and negative action values [26] , [27] , [28] , [29] , [45] . Absent any differences in overall task performance (easy contrast not significant), the presence of a DARPP-32 C allele was associated with an increased C>B bias in the conflict cost contrast (T/T N=35, T/C N=26, C/C N=22; t 82 =1.99, P =0.05), consistent with prior studies linking this allele to a bias towards reward-based learning and choice. This finding suggests that conflict acted to diminish striatal representations of reward value (B>C) in those who were more sensitive to reward/D1 learning (T alleles) and it acted to boost striatal representations of punishment avoidance (C>B) in those more sensitive to punishment/D2 learning (C alleles). Figure 5: A genetic polymorphism in dopamine receptors predicted individual differences in the cost of conflict on reward versus punishment. The presence of a DARPP-32 C allele was associated with an increased C>B bias in the conflict cost contrast ( t -test, N =83), bolstering the hypothesis that conflict diminished reward value (on the C stimulus) more in individuals biased to learn from reward and boosted punishment aversion (on the B stimulus) more in those biased to learn from punishment. Error bars are mean±s.e.m. * P =0.05. Full size image Study II participants and task Thirty participants were recruited from the Providence, RI community to participate in the double blind pharmacological study. Participants completed two experimental sessions no less than 1 week apart, with randomized double blind administration of either 1.25 mg of cabergoline or an identical looking placebo. Three participants were excluded from participation due to early adverse reactions of nausea and dizziness during their first session prior to this task (each of these three had cabergoline in the first session). This left a final sample of N =27 participants (mean age=20.5 years, range: 18–26 years; 12 female participants). The task was identical to Study I with one exception: the training RT deadline was diminished to 500 ms instead of 1,000 ms with the aim of boosting the effect of conflict during the training phase (with the intention of causing a greater cost of conflict to be revealed in the test phase, see Supplementary Fig. 4 ). We hypothesized that by reducing striatal dopamine, cabergoline would render learning and choices less driven by reward and more by punishment [30] , [31] , [32] , [33] , and hence would drive test phase action selection towards a C>B preference. Study II performance There were no reliable objective or subjective differences in physiology or feelings caused by the drug, and any idiosyncratic effects did not appear to be strong enough to reliably break the blind for the participants (see Online Methods). There were no effects of cabergoline in training phase performance. Consistent with the more stringent RT deadlines, participants had higher average error rates than Study I, but these were similar between sessions (placebo: 11%, s.d.=5%; cabergoline: 12%, s.d.=6%). Participants also had faster average congruent RT than in Study I, but these were still similar between sessions (placebo: 343 ms; cabergoline: 340 ms) with similarly small yet significant delays due to conflict (placebo: 12ms; cabergoline: 11 ms; main effect F 1,26 =35.53, P =3 e−6 ), see Fig. 6a . 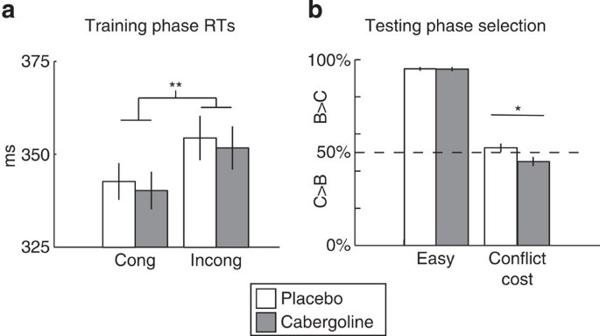Figure 6: Study II performance: cabergoline caused a selective bias to learn from punishment over reward, leading to an enhanced cost of conflict on punishment. (a) Training phase RT: a repeated measures analysis of variance (N=27) revealed a significant conflict effect in RT during Simon task performance, but no difference due to cabergoline. (b) Testing phase accuracies: whilet-tests did not reveal any difference in the easy condition, cabergoline caused a C>B conflict cost bias, suggesting that pre-synaptic agonism diminished reward learning (which would have favoured B>C) and boosted punishment learning (favouring C>B). Error bars are mean±s.e.m. *P<0.05; **P<0.01. Figure 6: Study II performance: cabergoline caused a selective bias to learn from punishment over reward, leading to an enhanced cost of conflict on punishment. ( a ) Training phase RT: a repeated measures analysis of variance ( N =27) revealed a significant conflict effect in RT during Simon task performance, but no difference due to cabergoline. ( b ) Testing phase accuracies: while t -tests did not reveal any difference in the easy condition, cabergoline caused a C>B conflict cost bias, suggesting that pre-synaptic agonism diminished reward learning (which would have favoured B>C) and boosted punishment learning (favouring C>B). Error bars are mean±s.e.m. * P <0.05; ** P <0.01. Full size image During the testing phase, RTs were nearly equivalent (placebo: 733ms, cabergoline: 731 ms) and participants were also nearly perfect when selecting A>D in the easy contrast (95% accuracy in each session). While the placebo session had small and non-significant numerical trends for biased B>C accuracy due to conflict ( t 26 =1.11, P =0.28), the effect of cabergoline was to reverse this bias towards avoidance (C>B). The difference between placebo and cabergoline was significant for the conflict cost contrast ( t 26 =−2.44, P =0.02), see Fig. 6b . Indeed, in the cabergoline session alone, participants had an opposing small and non-significant numerical trend for C>B ( t 26 =−1.97, P =0.06). There were no differences in EEG signals to conflict or feedback during training due to cabergoline ( Supplementary Fig. 5 ), consistent with our suggestion that cabergoline affected striatal but not cortical activities [30] . Study II spontaneous eye blink rate Spontaneous eye blink rate is thought to be a non-specific correlate of striatal dopaminergic tone [34] , [35] , [36] , [37] . We thus sought to examine whether cabergoline, as a dopaminergic agonist, would cause an alteration in blink rate, and if this alteration was tied to the hypothesized dopaminergic mediation of the cost of conflict. 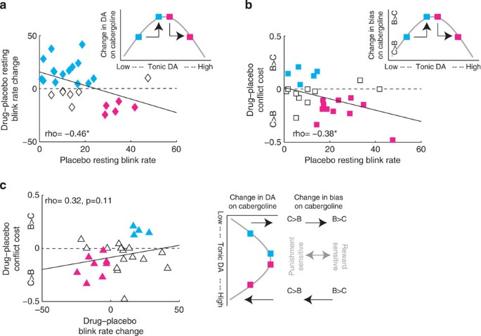Figure 7: Spontaneous eye blink rate at placebo predicted the valence-related shift in the cost of conflict under cabergoline. Some scatterplot icons are coloured to act as a visual cue linking the empirical data with the theorized underlying dopamine dynamics shown in the insets. (a) Placebo blink rate predicted a shift in blink rate change under cabergoline, consistent with an inverted-U effect. Inset: presumed cabergoline-induced shift in effective dopamine (DA) reflected by these measures. Higher blink rates are linked to higher tonic DA; for those with high DA, cabergoline primarily acts to reduce phasic DA, whereas for those with lower DA levels it can effectively have the opposite effect by stimulating unoccupied post-synaptic D2 receptors. (b) Placebo blink rate predicted whether cabergoline acts to increase conflict effects on punishment or reward. Inset: predicted shift in conflict effects on reward (cyan) versus punishment (magenta) sensitivities, according to presumed DA effects. High DA individuals (magenta) exhibit DA decreases under drug, causing conflict effects to predominate in punishment rather than reward, as revealed by the change in conflict cost bias. (c) Cabergoline-induced change in blink rate linearly related to the shift in the conflict cost bias (although non-significant). Inset: As suggested by the insets in (a,b), the cabergoline-induced change in DA and the change in conflict cost bias were linearly related. Correlations are Spearman’s rho onN=27 participants. *P<0.05. Figure 7a shows that cabergoline caused an inverted-U effect in blink rate: individuals with high blink rate at placebo had a lower rate under cabergoline, whereas those with a low placebo blink rate had an increase under cabergoline (rho 25 =−0.46, P =0.02). Importantly, baseline blink rate (in the placebo session) predicted the shift in the conflict cost bias due to cabergoline, where higher placebo blink rate (thus lower cabergoline blink rate) predicted a greater drug-induced bias towards conflict-induced punishment avoidance (rho 25 =−0.38, P =0.04). As should be expected from Fig. 7a,b , the cabergoline-induced blink rate change nearly predicted the conflict cost behavioural change (rho 25 =0.32, P =0.11). Similar (statistically significant) genetic, pharmacological and eye blink relationships were found using a related yet independent measure of the cost of conflict ( Supplementary Fig. 6 ). Figure 7: Spontaneous eye blink rate at placebo predicted the valence-related shift in the cost of conflict under cabergoline. Some scatterplot icons are coloured to act as a visual cue linking the empirical data with the theorized underlying dopamine dynamics shown in the insets. ( a ) Placebo blink rate predicted a shift in blink rate change under cabergoline, consistent with an inverted-U effect. Inset: presumed cabergoline-induced shift in effective dopamine (DA) reflected by these measures. Higher blink rates are linked to higher tonic DA; for those with high DA, cabergoline primarily acts to reduce phasic DA, whereas for those with lower DA levels it can effectively have the opposite effect by stimulating unoccupied post-synaptic D2 receptors. ( b ) Placebo blink rate predicted whether cabergoline acts to increase conflict effects on punishment or reward. Inset: predicted shift in conflict effects on reward (cyan) versus punishment (magenta) sensitivities, according to presumed DA effects. High DA individuals (magenta) exhibit DA decreases under drug, causing conflict effects to predominate in punishment rather than reward, as revealed by the change in conflict cost bias. ( c ) Cabergoline-induced change in blink rate linearly related to the shift in the conflict cost bias (although non-significant). Inset: As suggested by the insets in ( a , b ), the cabergoline-induced change in DA and the change in conflict cost bias were linearly related. Correlations are Spearman’s rho on N =27 participants. * P <0.05. Full size image In this report we provided evidence that response conflict implicitly influences reinforcement learning by acting as a cost that diminishes the value of reward and enhances aversion to punishment. Individual differences in cortical (FMθ) and striatal (DARPP-32) systems demonstrated how both of these areas contribute to the cost of conflict during reward and punishment learning. A direct manipulation of striatal dopamine via a selective D2 receptor agonist (cabergoline challenge) demonstrated that the cost of conflict can be selectively enhanced. Finally, an indirect measure of the resultant change in dopaminergic tone to drug challenge (blink rate) suggested that the degree of tonic dopaminergic diminishment predicted the resultant enhancement of the cost of conflict. Collectively, these findings validate prior hypotheses that conflict registers as a cost [1] , suggesting that the MCC evaluates the costs of effort, conflict and punishment in a similar manner [1] , [19] , [20] . These findings further suggest that this cost can manifest in terms of reduced reward value or enhanced punishment aversion, depending on the striatal dopaminergic state. The suggestion that conflict may act as a cost was motivated by a need to integrate two equally successful descriptions of MCC-related activities in the field of human EEG. Both conflict monitoring [46] , [47] and reinforcement learning [48] theories accurately accounted for ERP findings in a wealth of experiments. The conclusion that these theories were complementary rather than antagonistic was apparent, but a proposed common mechanism was required for theoretical integration. The study by Botvinick [1] suggested that if conflict monitoring was experienced to be aversive, then this would fit as a mediating construct between theories. We have similarly proposed that the MCC conflict detection mechanism could induce negative reward prediction, thereby driving avoidance [39] and that these previous ERP findings can be accounted for by a common FMθ mechanism reflecting MCC processes during the need for control [19] , [20] . The discoveries reported here provide evidence for each of these aforementioned theoretical integrations. Conflict and punishment were both specifically associated with 4–8 Hz enhancement, and power within this frequency range contributed to individual differences in the cost of conflict, whether by enhancing punishment aversion or by reducing reward values. One important implication of this finding is that individuals with larger FMθ conflict and error signals (such as in dispositional anxiety [21] , [49] ) may be more likely to discount the wilful tradeoff of difficulty for reward. Complementary supplementary analyses capitalized on the established but less well-known phenomenon of reward-related posterior delta band activities [19] , [42] . These additional findings demonstrate that while FMθ was commonly implicated in conflict-based alteration of both reward and punishment, similar effects are observable within a variety of cortical systems more specifically involved in assessing the salience of reinforcing events. If individual differences in MCC activities (that is, during training) contributed to the evaluation of reward and punishment values, the striatum was proposed to integrate these pieces of evidence to inform future action selection (that is, during testing). Individual differences in the tendency for effects to manifest in terms of reward or punishment were related to the DARPP-32 dopaminergic genotype that is relatively selective to striatum rather than cortex [50] and has been shown in the past to influence basic aspects of positive and negative learning [27] , [28] , [29] . Further evidence for a dopaminergic role in the cost of conflict was provided using a targeted pharmacological intervention of dopamine activities. Cabergoline is a selective D2 agonist, but in low doses this agent influences dopaminergic functioning in a manner contrary to common assumptions of receptor agonism. Low doses of D2 agonists reduce dopamine signalling by targeting pre-synaptic autoreceptors, diminishing phasic dopamine bursts and consequently decreasing reward learning and increasing relative learning from punishment [30] , [31] , [32] , [33] . Other studies have shown that low doses of cabergoline increase error awareness and response inhibition [51] , and cause a shift to a more conservative risk taking strategy [52] , all possibly due to a relative shift in indirect over direct pathway functioning. In the absence of nearly any other behavioural or EEG alteration, cabergoline caused a strong behavioural bias for C>B. This finding suggests that pre-synaptic agonism diminished reward responsiveness and boosted punishment responsiveness, causing conflict to have a relatively smaller influence on reward value (equivocating B and C rewards) and a larger influence on punishment aversion (boosting the aversion of B versus C punishments). Quantification of human striatal dopaminergic activities is challenging, yet we aimed to describe the robust pattern of effects caused by dopamine agonism using spontaneous eye blink rate, a controversial yet compelling candidate correlate of striatal dopaminergic tone [34] , [35] , [36] , [37] . Blink rates changed in a predictable inverted-U manner under cabergoline challenge as a function of baseline state, where high blink rate (putative high dopaminergic tone) under placebo predicted a diminishment under cabergoline (presumably lower dopaminergic tone) and vice versa for the other arm of the distribution. Placebo blink rate predicted the punishment-sensitive shift in the cost of conflict effect, with greater cabergoline-induced diminishment of blink rate predicting the largest shift in relative punishment sensitivity. A wealth of evidence from independent methods identified roles for medio–frontal cortex in the influence of conflict on reinforcement salience and striatum in the integration of conflict-altered reinforcement values to inform action selection. This effect could be manipulated using targeted dopaminergic challenge, and tracked via spontaneous eye blink rate. The proposed model of cortico–striatal interaction advanced here relies on examples from the field of effort-related discounting, as well as additional insight from computational modelling, the biology of striatal learning in opponent pathways and the modulation of these effects by dopamine. While many basic features of cortico–striatal systems are increasingly well-defined, it remains a challenge to empirically describe the combined interaction of these processes. In summary, conflict appears to act as a cost in reinforcement learning in a manner similar to effort, punishment and errors. This finding provides evidence for the suggestion that the MCC uses a common process for interpreting the averseness of events requiring a need for control [1] , and further supports the theory that FMθ reflects these general MCC operations [19] , [20] . Participants Both experiments were approved by the Brown University Institutional Review Board and all participants provided written informed consent. All participants had normal or corrected-to-normal vision, no history of neurological, psychiatric, or any other relevant medical problem, and were free from current psychoactive medication use. For Study I, participants received either course credit or $20 for participation. For Study II, participants were paid $40 for the first session and $60 for the second session. Study II also had the additional inclusion criteria that women were required to be on birth control or not be sexually active. After drug or placebo administration, participants began the task described here at an average of 2 h 22 min following ingestion (range: 2 h 5 min to 2 h 45 min). This task took an average of 37 min (range: 31 to 50 min) to complete. Statistical analyses There was no way to determine an a priori sample size as the effect size of the cost of conflict was unknown. Study I aimed to match previous sample sizes of genetic studies from this lab, for instance the study by Doll et al. [28] had N =80 (here we had N =83). Study II used the same target as the previous cabergoline study of the Principal Investigator (PI) (ref. 30 ), which had N =28 (here we ran N =30 expecting some dropout). For Study I, two-tailed t -tests ( Figs 2 , 3 and 5 ), Spearman’s rho ( Fig. 4 ), and two-tailed z -tests of the rho-to- z converted coefficients ( Fig. 4 ) were used. For Study II, repeated measures analysis of variance, t -tests ( Fig. 6 ), and Spearman’s rho ( Fig. 7 ) were used. Skewness was tested prior to t -tests: all measures of skew were <0.25. In Study II, participants were randomly assigned to a drug or placebo condition (that is, drug first versus second visit) based on a random-number generated table. The experimenter (S.E.M.) did not have the key describing which session each participant was in: the pills were set up by J.F.C. who alone had the key and did not interact with the subjects. EEG recording and preprocessing EEG was recorded continuously across 0.1–100 Hz with a sampling rate of 500 Hz and an online CPz reference on a 64-channel Brain Vision system. Data were then epoched around the cues (−1,500 to 5,000 ms), from which the associated responses and feedbacks were isolated. CPz was re-created and data were then visually inspected to identify bad channels to be interpolated, and bad epochs to be rejected. Time-frequency measures were computed by multiplying the fast Fourier transformed (FFT) power spectrum of single trial EEG data with the FFT power spectrum of a set of complex Morlet wavelets (defined as a Gaussian-windowed complex sine wave: , where t is time, f is frequency (which increased from 1–50 Hz in 50 logarithmically spaced steps), and defines the width (or ‘cycles’) of each frequency band, set according to 4/(2 πf )), and taking the inverse FFT. The end result of this process is identical to time-domain signal convolution, and it resulted in estimates of instantaneous power (the magnitude of the analytic signal), defined as Z[ t ] (power time series: p( t )=real[z( t )] 2 +imag[z( t )] 2 ). Each epoch was then cut in length (−500 to +1,000 ms). Power was normalized by conversion to a decibel scale (10 × log10[power( t )/power(baseline)]), allowing a direct comparison of effects across frequency bands. The baseline for each frequency consisted of the average power from −300 to −200 ms prior to the onset of the cues. For Fig. 3 , paired t -tests were used to determine statistical significance with a cluster-based threshold of 500 pixels applied to the significant contrasts. Since a wealth of work from our lab and others have demonstrated that pre-response conflict and post-feedback punishment effects are most strongly represented in the 4–8 Hz range, these strongly justified that a priori region-of-interests preclude the need for extensive formal multiple comparison testing. ERPs were created from each epoch and then filtered from 0.5–20 Hz in two steps using the EEGLab function eegfilt. Response-locked ERPs were quantified as the mean value from −70 to −50 ms pre-response (congruent M =−0.02, s.d.=0.08; incongruent M =0.006, s.d.=0.09). Feedback-locked ERPs were quantified as the mean value from 200 to 300 ms after feedback (correct M =0.14, s.d.=0.10; incongruent M =0.12, s.d.=0.10). DNA extraction and genotypic analysis Genomic DNA was collected and purified for genetic analysis using the manufacturer’s protocol. For genotyping, we used Taqman 5′ exonuclease assays (ABI) for the rs907094 (DARPP-32) SNP. Assays were performed on a CFX384 apparatus (Biorad) in real-time PCR mode using standardized cycling parameters for ABI Assays on Demand. Fluorescence was then analyzed using the allelic discrimination function in the CFX software. Amplification curves were visually inspected for each of the assays that led to determination of the genotype. All samples were required to give clear and concordant results and all samples that did not were re-run and/or re-extracted until they provided clear genotype calls. Cabergoline side effects Measurements of blood pressure, heart rate and self-reported feelings were taken at four times throughout the experiment: (1) immediately following administration (baseline), (2) 1 h following administration, (3) 2 h 20 min following administration (immediately prior to this experiment), and (4) an average of 1 h 8 min following time point #3 (after this experiment and another were finished). There were no group differences in physiological changes from the baseline measure, nor were there meaningful changes in self-reported feelings, as the median responses were identical between groups in most cases. On the final rating form (time point #4 above), participants were asked to rate their confidence that they received the drug in this session. Although the drug group had slightly higher confidence ratings, there was no significant difference between groups ( t 25 =1.53, P =0.14). Spontaneous blink rate For assessment of spontaneous eye blink rate, vertical electro-oculogram (VEOG) recordings were taken from 2 min of resting EEG data gathered prior to all tasks. Two independent evaluators counted blinks from VEOG. If there was any disagreement, a third evaluator counted the blinks and the per-minute rate was quantified as the average of the two closest scores. Correlations between raters exceeded r =0.97. How to cite this article: Cavanagh, J. F. et al. Conflict acts as an implicit cost in reinforcement learning. Nat. Commun. 5:5394 doi: 10.1038/ncomms6394 (2014).